Anomalous critical fields in quantum critical superconductors Fluctuations around an antiferromagnetic quantum critical point (QCP) are believed to lead to unconventional superconductivity and in some cases to high-temperature superconductivity. However, the exact mechanism by which this occurs remains poorly understood. The iron-pnictide superconductor BaFe 2 (As 1− x P x ) 2 is perhaps the clearest example to date of a high-temperature quantum critical superconductor, and so it is a particularly suitable system to study how the quantum critical fluctuations affect the superconducting state. Here we show that the proximity of the QCP yields unexpected anomalies in the superconducting critical fields. We find that both the lower and upper critical fields do not follow the behaviour, predicted by conventional theory, resulting from the observed mass enhancement near the QCP. Our results imply that the energy of superconducting vortices is enhanced, possibly due to a microscopic mixing of antiferromagnetism and superconductivity, suggesting that a highly unusual vortex state is realized in quantum critical superconductors. Quantum critical points (QCPs) can be associated with a variety of different order–disorder phenomena, however, so far superconductivity has only been found close to magnetic order. Superconductivity in heavy fermions, iron pnictides and organic salts is found in close proximity to antiferromagnetic order [1] , [2] , whereas in the cuprates the nature of the order (known as the pseudogap phase) is less clear [3] . The normal state of these materials has been widely studied and close to their QCPs non-Fermi liquid behaviour of transport and thermodynamic properties are often found, however, comparatively little is known about how the quantum critical fluctuations affect the superconducting state [4] . This is important as it is the difference in energy between the normal and superconducting state that ultimately determines the critical temperature T c . Among the various iron-pnictide superconductors, BaFe 2 (As 1− x P x ) 2 has proved to be the most suitable family for studying the influence of quantum criticality on the superconducting state. This is because the substitution of As by P introduces minimal disorder as it tunes the material across the phase diagram from a spin-density wave antiferromagnetic metal, through the superconducting phase to a paramagnetic metal [5] . The main effect is a compression of the c axis arising from the smaller size of the P ion compared with As, which mimics the effect of external pressure [6] . Normal state properties such as the temperature dependence of the resistivity [7] and spin-lattice relaxation rate [8] clearly point to a QCP at x =0.30. Measurements of superconducting state properties that show signatures of quantum critical effects include the magnetic penetration depth λ and the heat capacity jump at T c , Δ C [9] , [10] . Both of these quantities show a strong increase as x tends to 0.30, and it is shown that this could be explained by an underlying approximately sixfold increase in the quasiparticle effective mass m * at the QCP [10] . In the standard single-band Ginzburg–Landau theory, the upper critical field is given by where φ 0 is the flux quantum and ξ GL is the Ginzburg–Landau coherence length. In the clean limit at low temperature, ξ GL is usually well approximated by the BCS coherence length, which results in H c2 ∝ ( m *Δ) 2 , where m * is the mass of the quasiparticles and Δ is the superconducting gap. This simplified analysis is borne out by the full strong coupling BCS theory [11] . Hence, a strong peak in m * at the QCP should result in a corresponding increase in H c2 as well as the slope of H c2 at . This latter quantity is often more easily accessible experimentally because of the very high H c2 values in compounds such as iron pnictides for T ≪ T c and also because the values of H c2 close to T c are not reduced by the effect of the magnetic field on the electron spin (Pauli limiting effects). For the lower critical field H c1 , standard Ginzburg–Landau theory predicts that where κ = λ / ξ GL , and so the observed large peak in λ at the QCP [9] should result in a strong suppression of H c1 . Here we show that the exact opposite, a peak in H c1 at the QCP, occurs in BaFe 2 (As 1− x P x ) 2 , and in addition the expected sharp increase in H c2 is not observed. This suggests that the critical fields of quantum critical superconductors strongly violate the standard theory. Upper critical field H c2 We measured H c2 parallel to the c axis, in a series of high-quality single-crystal samples of BaFe 2 (As 1− x P x ) 2 spanning the superconducting part of the phase diagram using two different techniques. Close to T c ( H =0), we measured the heat capacity of the sample using a microcalorimeter in fields up to 14 T (see Fig. 1a ). This gives an unambiguous measurement of H c2 ( T ) and the slope h ′, which unlike transport measurements is not complicated by contributions from vortex motion [12] . At a lower temperature, we used micro-cantilever torque measurements in pulsed magnetic fields up to 60 T. Here an estimate of H c2 was made by observing the field where hysteresis in the torque magnetization loop closes (see Fig. 1b ). Although, strictly speaking, this marks the irreversibility line H irr , this is a lower limit for H c2 (0) and in superconductors with negligible thermal fluctuations and low anisotropy such as BaFe 2 (As 1− x P x ) 2 H irr should coincide approximately with H c2 . Indeed, in Fig. 2 we show that the extrapolation of the high-temperature-specific heat results, using the Helfand–Werthamer (HW) formula [13] , to zero temperature are in good agreement with the irreversibility field measurements showing both are good estimates of H c2 (0). 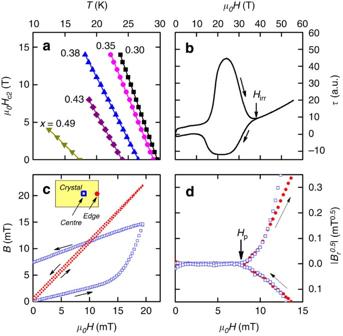Figure 1: Determination of critical fields. (a)Hc2(T) data close toTc(H=0) from heat capacity measurements for different samples of BaFe2(As1−xPx)2. (b) Magnetic torque versus rising and falling field for a sample withx=0.40 atT=1.5 K. The irreversibility fieldHirris marked. (c) Magnetic flux densityBversus applied fieldHas measured by the micro-Hall sensors, forx=0.35 andT=18 K at two different sensor positions: one at the edge of the sample and the other close to the centre (schematic inset). (d) Remnant fieldBrafter subtraction of the linear term due to flux leakage around the sample. |Br|0.5versusμ0His plotted as this best linearizesBr(H)14. Note that the changes in linearity ofB(H) evident indare not visible by eye inc. Figure 1: Determination of critical fields. ( a ) H c2 ( T ) data close to T c ( H =0) from heat capacity measurements for different samples of BaFe 2 (As 1− x P x ) 2 . ( b ) Magnetic torque versus rising and falling field for a sample with x =0.40 at T =1.5 K. The irreversibility field H irr is marked. ( c ) Magnetic flux density B versus applied field H as measured by the micro-Hall sensors, for x =0.35 and T =18 K at two different sensor positions: one at the edge of the sample and the other close to the centre (schematic inset). ( d ) Remnant field B r after subtraction of the linear term due to flux leakage around the sample. | B r | 0.5 versus μ 0 H is plotted as this best linearizes B r ( H ) [14] . Note that the changes in linearity of B ( H ) evident in d are not visible by eye in c . 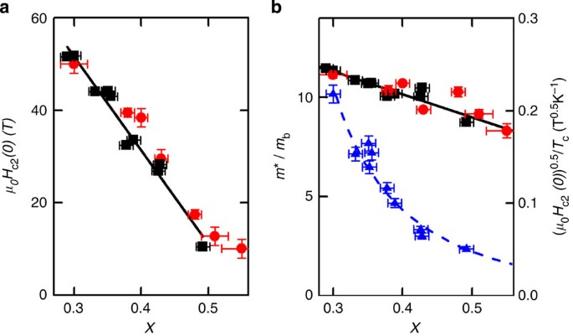Figure 2: Upper critical field as a function of concentrationx. (a)Hc2(0) in BaFe2(As1−xPx)2estimated from the slope ofHc2(T) close toTcusing(squares)13, and also estimates ofHc2(0) from the irreversibility field at low temperature (T=1.5 K) measured by torque magnetometry (circles). Error bars onHc2(circles) represent the uncertainties in locatingHirrand (squares) in extrapolating the values close toTctoT=0. Error bars onxrepresent s.d. (b) The same data plotted as (Hc2(0))0.5/Tc, which, in conventional theory, are proportional to the mass enhancementm*. The mass renormalizationm*/mbderived from specific heat measurements is shown for comparison (triangles)10. The dashed line is a guide to the eye and solid lines in both parts are linear fits to the data. Full size image Figure 2: Upper critical field as a function of concentration x . ( a ) H c2 (0) in BaFe 2 (As 1− x P x ) 2 estimated from the slope of H c2 ( T ) close to T c using (squares) [13] , and also estimates of H c2 (0) from the irreversibility field at low temperature ( T =1.5 K) measured by torque magnetometry (circles). Error bars on H c2 (circles) represent the uncertainties in locating H irr and (squares) in extrapolating the values close to T c to T =0. Error bars on x represent s.d. ( b ) The same data plotted as ( H c2 (0)) 0.5 / T c , which, in conventional theory, are proportional to the mass enhancement m *. The mass renormalization m */ m b derived from specific heat measurements is shown for comparison (triangles) [10] . The dashed line is a guide to the eye and solid lines in both parts are linear fits to the data. Full size image In the clean limit we would expect ( H c2 (0)) 1/2 / T c to be proportional to the renormalized effective mass m *. Surprisingly, we show in Fig. 2 that this quantity increases by just ~20% from x =0.47 to x =0.30, whereas m * increases by ~400% for the same range of x . Lower critical field H c1 We measured H c1 in our BaFe 2 (As 1− x P x ) 2 samples using a micro-Hall probe array. Here the magnetic flux density B is measured at several discrete points a few microns from the surface of the sample. Below H c1 , B increases linearly with the applied field H due to incomplete shielding of the sensor by the sample. Then, as the applied field passes a certain field H p , B increases more rapidly with H indicating that vortices have entered the sample (see Fig. 1c,d ). Care must be taken in identifying H p with H c1 because, in some cases, surface pinning and geometrical barriers can push H p well above H c1 . However, in our measurements, several different checks, such as the equality of H p for increasing and decreasing field [14] , and the independence of H p on the sensor position [15] , rule this out (see Methods). The temperature dependence of H c1 is found to be linear in T at low temperature for all x ( Fig. 3 ), which again is indicative of a lack of surface barriers that tend to become stronger at low temperature causing an upturn in H c1 ( T ) [16] . Extrapolating this linear behaviour to zero temperature gives us H c1 (0), which is plotted versus x in Fig. 4a . Surprisingly, instead of a dip in H c1 (0) at the QCP predicted by equation (2) in conjunction with the observed behaviour of λ ( x ) [9] , there is instead a strong peak. To resolve this discrepancy we consider again the arguments leading to equation (2). 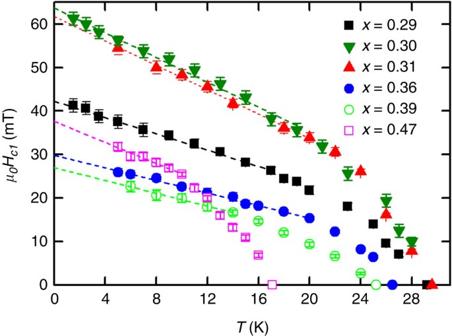Figure 3: Temperature dependence ofHc1in samples of BaFe2(As1−xPx)2. The lines show the linear extrapolation used to determine the value atT=0. Error bars represent the uncertainty in locatingHc1from the rawB(H) data. Figure 3: Temperature dependence of H c1 in samples of BaFe 2 (As 1− x P x ) 2 . The lines show the linear extrapolation used to determine the value at T =0. Error bars represent the uncertainty in locating H c1 from the raw B ( H ) data. 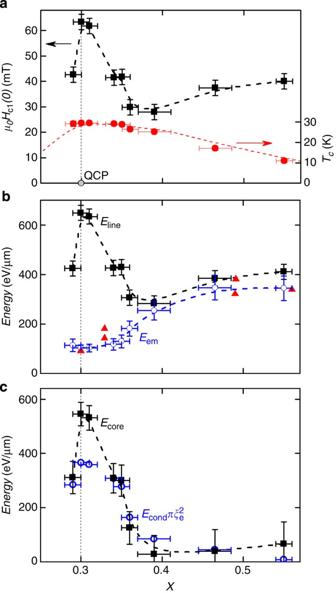Figure 4: Concentrationxdependence of lower critical field and associated energies for BaFe2(As1−xPx)2. (a) Lower critical fieldHc1extrapolated toT=0 andTc. The location of the QCP is indicated. Error bars onHc1represent the combination of uncertainties in extrapolatingHc1(T) toT=0 and in the demagnetizing factor. Error bars onxare s.d. (b) Vortex line energyEline=Eem+EcoreatT=0 from theHc1(0) data and equations (4) and (3) shown as squares. The electromagnetic energy calculated using equation (4) and different estimates ofλare also shown. The triangles are direct measurements from ref.9, and the circles are estimates derived by scaling the band-structure value ofλby the effective mass enhancement from specific heat10. Error bars onEem(circles) are calculated from the uncertainty in jump size in heat capacity atTc. (c) Vortex core energyEcore=Eline−Eemalong with an alternative estimate derived from the specific heat condensation energy (Econd) and the effective vortex area (πξe2). The uncertainties are calculated from a combination of those in the other panels. The dashed lines in all panels are guides to the eye. Full size image Figure 4: Concentration x dependence of lower critical field and associated energies for BaFe 2 (As 1− x P x ) 2 . ( a ) Lower critical field H c1 extrapolated to T =0 and T c . The location of the QCP is indicated. Error bars on H c1 represent the combination of uncertainties in extrapolating H c1 ( T ) to T =0 and in the demagnetizing factor. Error bars on x are s.d. ( b ) Vortex line energy E line = E em + E core at T =0 from the H c1 (0) data and equations (4) and (3) shown as squares. The electromagnetic energy calculated using equation (4) and different estimates of λ are also shown. The triangles are direct measurements from ref. 9 , and the circles are estimates derived by scaling the band-structure value of λ by the effective mass enhancement from specific heat [10] . Error bars on E em (circles) are calculated from the uncertainty in jump size in heat capacity at T c . ( c ) Vortex core energy E core = E line − E em along with an alternative estimate derived from the specific heat condensation energy ( E cond ) and the effective vortex area ( πξ e 2 ). The uncertainties are calculated from a combination of those in the other panels. The dashed lines in all panels are guides to the eye. Full size image In general H c1 is determined from the vortex line energy E line , which is composed of two parts [17] , The first, E em is the electromagnetic energy associated with the magnetic field and the screening currents, which in the high κ approximation is given by The second contribution arises from the energy associated with creating the normal vortex core E core . In high κ superconductors, E core is usually almost negligible and is accounted for by the additional constant 0.5 in equation (2). However, in superconductors close to a QCP we argue this may not be the case. In Fig. 4b,c we use equations (3) and (4) to determine E em and E core . Away from the QCP, E core is approximately zero and so the standard theory accounts for H c1 (0) well. However, as the QCP is approached there is a substantial increase in E core as determined from the corresponding increase in H c1 . We can check this interpretation by making an independent estimate of the core energy from the condensation energy E cond , which we estimate from the experimentally measured specific heat (see Methods). The core energy is then , where ξ e is the effective core radius that may be estimated from the coherence length ξ GL derived from H c2 measurements using equation (1). In Fig. 4 , we see that has a similar dependence on x as E core and is in approximate quantitative agreement if ξ e ≅ 4.0 ξ GL for all x . Hence, this suggests that the observed anomalous increase in H c1 could be caused by the high energy needed to create a vortex core close to the QCP. In principle, the relative lack of enhancement in H c2 close to the QCP could be caused by impurity or multiband effects, although we argue that neither are likely explanations. Impurities decrease ξ GL and in the extreme dirty limit H c2 ∝ m * T c / ℓ , where ℓ is the electron mean-free-path [11] . Hence, even in this limit we would expect H c2 to increase with m * although not as strongly as in the clean case. Impurities increase H c2 and as the residual resistance increases close to x =0.3 (ref. 7 ) we would actually expect a larger increase in H c2 than expected from clean-limit behaviour. dHvA measurements show that ℓ >> ξ GL at least for the electron bands and for x >0.38, which suggest that, in fact, our samples are closer to the clean limit. To discuss the effect of multiple Fermi surface sheets on H c2 , we consider the results of Gurevich [18] for two ellipsoidal Fermi surface sheets with strong interband pairing. This limit is probably the one most appropriate for BaFe 2 (As 1− x P x ) 2 (ref. 19 ). In this case for H || c , were υ 1,2 are the in-plane Fermi velocities on the two sheets. So if the velocity was strongly renormalized on one sheet only ( υ 1 →0) then H c2 would be determined mostly by υ 2 on the second sheet and hence would not increase with m * in accordance with our results. However, in this case the magnetic penetration depth λ , which will also be dominated by the Fermi surface sheet with the largest υ , would not show a peak at the QCP in disagreement with experiment [9] . In fact, the numerical agreement between the increase in m * with x as determined by λ or specific heat, which in contrast to λ is dominated by the low Fermi velocity sections, rather suggests that the renormalization is mostly uniform on all sheets [10] . In the opposite limit, appropriate to the prototypic multiband superconductor MgB 2 , where intraband pairing dominates over interband, H c2 will be determined by the band with the lowest υ (ref. 18 ) and again an increase in m * should be reflected in H c2 . So these multiband effects cannot easily explain our results. Another effect of multiband superconductivity is that it can modify the temperature dependence of H c2 such that it departs from the HW model. For example, in some iron-based superconductors a linear dependence of H c2 ( T ) was found over a wide temperature range [20] . For BaFe 2 (As 1− x P x ) 2 , however, the coincidence between the HW extrapolation of the H c2 data close to T c and the pulsed field measurement of H irr for T ≪ T c for all x , would appear to rule out any significant underestimation of H c2 (0). In Supplementary Fig. 3 we show that H irr for a sample with x =0.51 fits the HW theory for H c2 ( T ) over the full temperature range. There is no reason why H irr would underestimate H c2 (0) by the same factor as the HW extrapolation. Even in cuprate superconductors where, unlike here, there is evidence for strong thermal fluctuation effects, H irr has been shown to agree closely with H c2 in the low-temperature limit [21] . The magnitude of the discrepancy between the behaviour of H c2 (0) and m * discussed above (see Fig. 2 ) also makes an explanation based on an experimental underestimate of H c2 (0) implausible. Another possibility is that in heavy fermion superconductors the mass enhancement is often reduced considerably at high fields and therefore m * could be reduced at fields comparable to H c2 . In BaFe 2 (As 1− x P x ) 2 , however, a significantly enhanced mass in fields greater than H c2 can be inferred from the dHvA measurements [10] and low temperature, high field, resistivity [22] . Although very close to the QCP the mass inferred from these measurements is slightly reduced from the values inferred from the zero field specific heat measurements [10] this cannot account for the lack of enhancement of H c2 shown in Fig. 2 . Our results are similar to the behaviour observed in another quantum critical superconductor, CeRhIn 5 . Here the pressure tuned QCP manifests a large increase in the effective mass as measured by the dHvA effect and the low-temperature resistivity. T c is maximal at the QCP but H c2 displays only a broad peak, inconsistent with the mass enhancement shown by the other probes [23] . We should note that in this system H c2 at low temperatures is Pauli limited. However, close to T c , H c2 is always orbitally limited and as neither h ′ or H c2 (0) are enhanced in BaFe 2 (As 1− x P x ) 2 or CeRhIn 5 (ref. 23 ), Pauli limiting can be ruled out as the explanation. A comparison with the behaviour observed in cuprates is also interesting. Here two peaks in H c2 (0) as a function of doping p in YBa 2 Cu 3 O 7− δ have been reported [21] , which approximately coincide with critical points where other evidence suggests that the Fermi surface reconstructs. Quantum oscillation measurements indicate that m * increases close to these points [24] , suggesting a direct link between H c2 (0) and m * in the cuprates in contrast to our finding here for BaFe 2 (As 1− x P x ) 2 . However, by analysing the data in the same way as we have done here, it can be seen [25] that H c2 (0) 0.5 / T c for YBa 2 Cu 3 O 7− δ is independent of p above p ≅ 0.18 and falls for p below this value, reaching a minimum at p ≅ 1/8. This suggests that at least the peak at higher p is driven by the increasing gap value rather than a peak in m *, in agreement with our results here, and that the minimum in H c2 (0) 0.5 / T c coincides with the doping where charge order is strongest at p ≅ 1/8 (ref. 26 ). The lack of enhancement of H c2 (0) in all these systems suggests a fundamental failure of the theory. One possibility is that this may be driven by microscopic mixing of superconductivity and antiferromagnetism close to the QCP. In the vicinity of the QCP, antiferromagnetic order is expected to emerge near the vortex core region where the superconducting order parameter is suppressed [27] , [28] . Such a field-induced antiferromagnetic order has been observed experimentally in cuprates [29] , [30] . When the QCP lies beneath the superconducting dome, as in the case of BaFe 2 (As 1− x P x ) 2 (refs 4 , 9 ), antiferromagnetism and superconductivity can coexist on a microscopic level. In such a situation, as pointed out in ref. 28 , the field-induced antiferromagnetism can extend outside the effective vortex core region where the superconducting order parameter is finite. Such an extended magnetic order is expected to lead to further suppression of the superconducting order parameter around vortices. This effect will enlarge the vortex core size, which in turn will suppress the upper critical field in agreement with our results. We would expect this effect to be a general feature of superconductivity close to an antiferromagnetic QCP, but perhaps not relevant to the behaviour close to p =0.18 in the cuprates. To explain the H c1 results we postulate that the vortex core size is around four times larger than the estimates from H c2 . This is in fact expected in cases of multiband superconductivity or superconductors with strong gap anisotropy. In MgB 2 (refs 31 , 32 ) and also in the anisotropic gap superconductor 2 H -NbSe 2 (ref. 33 ) the effective core size has been found to be around three times ξ GL , similar to that needed to explain the behaviour here. BaFe 2 (As 1− x P x ) 2 is known to have a nodal gap structure [34] , which remains relatively constant across the superconducting dome [9] and so we should expect the core size to be uniformly enhanced for all x . The peak in H c1 ( x ) at the QCP is then, primarily caused by the fluctuation-driven enhancement in the normal-state energy, but the effect is magnified by the nodal gap structure of BaFe 2 (As 1− x P x ) 2 . We expect the observed anomalous increase in H c1 to be a general feature of quantum critical superconductors as these materials often have nodal or strongly anisotropic superconducting gap structures and the increase in normal state energy is a general property close to a QCP. The relative lack of enhancement in H c2 also seems to be a general feature, which may be linked to a microscopic mixing of antiferromagnetism and superconductivity. Sample growth and characterization BaFe 2 (As 1− x P x ) 2 samples were grown using a self-flux technique as described in ref. 7 . Samples for this study were screened using specific heat and only samples with superconducting transition width <1 K were measured (see Supplementary Fig. 1 ). To determine the phosphorous concentration in the samples we carried out energy-dispersive X-ray analysis on several randomly chosen spots on each crystal ( H c1 samples) or measured the c axis lattice parameter using X-ray diffraction ( H c2 samples), which scales linearly with x . For some of the H c2 samples measured using high-field torque magnetometry the measured de Haas–van Alphen frequency was also used to determine x as described in ref. 10 . Measurements of H c2 Close to T c the upper critical field was determined using heat capacity. For this a thin film microcalorimeter was used [10] . We measured the superconducting transition at constant magnetic field up to 14 T (see Supplementary Fig. 2 ). The midpoint of the increase in C at the transition defines T c ( H ). At low temperatures ( T ≪ T c ) we used piezo-resistive microcantilevers to measure the magnetic torque in pulsed magnetic field and hence determine the irreversibility field H irr . The crystals used in the pulsed field study were the same as those used in ref. 10 for the de Haas–van Alphen effect (except samples for x ≅ 0.3). By taking the difference between the torque in increasing and decreasing field we determined the point at which the superconducting hysteresis closes as H irr (see Fig. 1b ). For some compositions we measured H irr in d.c. field over the full temperature range and found it to agree well with the HW model and also the low-temperature measurements in pulsed field on the same sample ( Supplementary Fig. 3 ). Our heat capacity measurements of H c2 close to T c ( H =0) are in good agreement with those of ref. 35 . Measurements of H c1 The measurements of the field of first flux penetration H p have been carried out using micro-Hall arrays. The Hall probes were made with either GaAs/AlGaAs heterostructures (carrier density n s =3.5 × 10 11 cm −2 ) or GaAs with a 1 μm thick silicon doped layer (concentration n s =1 × 10 16 cm −3 ). The latter had slightly lower sensitivity but proved more reliable at temperatures below 4 K. The measurements were carried out using a resistive magnet so that the remanent field during zero field cooling was as low as possible. The samples were warmed above T c after each field sweep and then cooled at a constant rate to the desired temperature. When strong surface pinning is present H p may be pushed up significantly beyond H c1 . In this case there will also be a significant difference between the critical field H p measured at the edge and the centre of the sample (for example see ref. 15 ) and also a difference between the field where flux starts to enter the sample and the field at which it leaves. Some of our samples, also showing signs of inhomogeneity, such as wide superconducting transitions, showed this behaviour. An example is shown in Supplementary Fig. 4 . In this sample the sensor at the edge shows first flux penetration at H p ≈5 mT, whereas the value is ~3 times higher at the centre. For decreasing fields, the centre sensor shows a similar value to the edge sensor. All the samples reported in this paper showed insignificant difference between H p at the centre and the edge and also for increasing and decreasing fields. Hence, we conclude that H c1 in our samples is not significantly increased by pinning. As our samples are typically thin platelets, demagnetization effects need to be taken into account for measurement of H c1 . Although an exact solution to the demagnetization problem is only possible for ellipsoids and infinite slabs, a good approximation for thin slabs has been obtained by Brandt [36] . Here H c1 is related to the measured H p , determined from H using where l c is the sample dimension along the field and l a perpendicular to the field. All samples in this study had l c ≪ l a . To ensure that the determination of the effective field is independent of the specific dimension we have carried out multiple measurements on a single sample cleaved to give multiple ratios of l c / l a . The results of this study ( Supplementary Fig. 5 ) show that H c1 determined by this method are independent of the aspect ratio of the sample. Furthermore, the samples used all had similar l c / l a ratios (see Supplementary Table 1 ), and so any correction would not give any systematic errors as a function of x . Calculation of condensation energy The condensation energy can be calculated from the specific heat using the relation To calculate this, we first measured a sample of BaFe 2 (As 1− x P x ) 2 with x =0.47, using a relaxation technique in zero field and μ 0 H =14 T, which is sufficient at this doping to completely suppress superconductivity and thus reach the normal state. We used this 14 T data to determine the phonon heat capacity and we then subtract this from the zero field data to give the electron specific heat of the sample. We then fitted this data to a phenomenological nodal gap, alpha model (with variable zero temperature gap) similar to that described in ref. 37 (see Supplementary Fig. 6 ). We then integrated this fit function using equation (6) to give E cond for this value of x . For lower values of x (higher T c ) the available fields were insufficient to suppress superconductivity over the full range of temperature, so we assumed that the shape of the heat capacity curve does not change appreciably with x but rather just scales with T c and the jump height at T c . This is implicitly assuming that the superconducting gap structure does not change appreciably with x , which is supported by magnetic penetration depth λ measurements which show that normalized temperature dependence λ ( T )/ λ (0) is relatively independent of x [9] . With this assumption we can then calculate where x ref =0.47. How to cite this article: Putzke, C. et al. Anomalous critical fields in quantum critical superconductors. Nat. Commun. 5:5679 doi: 10.1038/ncomms6679 (2014).